DNA repair choice defines a common pathway for recruitment of chromatin regulators DNA double-strand break repair is essential for maintenance of genome stability. Recent work has implicated a host of chromatin regulators in the DNA-damage response, and although several functional roles have been defined, the mechanisms that control their recruitment to DNA lesions remain unclear. Here we find that efficient double-strand break recruitment of the INO80, SWR-C, NuA4, SWI/SNF and RSC enzymes is inhibited by the non-homologous end-joining machinery, and that their recruitment is controlled by early steps of homologous recombination. Strikingly, we find no significant role for H2A.X phosphorylation in the recruitment of chromatin regulators, but rather their recruitment coincides with reduced levels of H2A.X phosphorylation. Our work indicates that cell cycle position has a key role in DNA repair pathway choice and that recruitment of chromatin regulators is tightly coupled to homologous recombination. Cell viability and genomic stability are frequently threatened by chromosomal DNA double-strand breaks (DSBs). DSBs can be induced by endogenous free oxygen radicals, collapsed replication forks or exposure to DNA-damaging agents, such as ionizing radiation, ultraviolet light and chemicals [1] . The failure or improper repair of DSBs can result in cell death or gross chromosomal changes, including deletions, translocations and fusions that promote genome instability and tumorigenesis [2] . Consequently, cells have developed complex signalling networks that sense DSBs, arrest the cell cycle and activate the repair pathways. Eukaryotic cells have evolved two major mechanisms that repair chromosomal DSBs, non-homologous end joining (NHEJ) and homologous recombination (HR). NHEJ is the predominant DSB repair mechanism in the G1 phase of the cell cycle, whereas HR predominates in the S and G2 phases [3] , [4] , [5] , [6] , [7] . In the case of NHEJ, the broken DNA ends are recognized and bound by the Ku70/Ku80 heterodimer, which subsequently recruits other factors to facilitate ligation of the ends [8] , [9] , [10] . In contrast, DSB repair by HR relies on sequence homology from an undamaged sister chromatid or a homologous DNA sequence to use as a template for copying the missing information. The first step of HR involves extensive processing of the DSB such that the 5′ ends of the DNA duplex that flank the DSB are resected to generate long, 3′ single-stranded tails [11] . Notably, extensive processing of the DSB ends is inhibited in G1 phase cells by the Ku70/80 complex [7] , and increased CDK activity at the G1/S boundary activates DSB processing during later cell cycle phases [4] , [5] , [12] . DSB processing regulates the differential recruitment of two functionally related, checkpoint kinases ATM and ATR (Tel1 and Mec1, respectively in budding yeast). ATM recruitment does not require extensive DSB processing, whereas recruitment of the ATR/ATRIP (scMec1/Ddc2) checkpoint kinase complex requires the binding of the single-stranded binding protein replication protein A (RPA) to the processed DNA [13] , [14] . One of the most intensively studied targets for checkpoint kinases is the histone variant H2A.X, which is phosphorylated at a C-terminal serine residue (H2A S129 in yeast or H2A.X S139 in higher eukaryotes; termed H2A.X phosphorylation (γH2AX)). The formation of γH2AX is one of the earliest events at a DSB, and this mark spreads over at least a megabase of chromatin adjacent to each DSB in mammalian cells, and up to 50 kb on each side of a DSB in budding yeast [15] , [16] . Although γH2AX is not essential for the initial recruitment of DSB response factors, it has a role in stabilizing the binding of checkpoint factors to DSB chromatin [17] . Besides its role in the DNA-damage checkpoint, γH2AX has also been proposed to recruit chromatin-regulatory factors, namely the ATP-dependent chromatin remodelling complexes INO80 and SWR-C [18] , [19] . These results have established γH2AX as both a ubiquitous hallmark and regulator of the chromatin response to DSBs. In budding yeast, the DSB recruitment of chromatin regulators has been monitored primarily in asynchronous cell populations, and thus it is unclear if these events are linked to NHEJ or HR. To investigate whether the chromatin response to DNA damage is defined by a specific DSB repair pathway, we induced a single DSB within yeast cells synchronized in either G1 or G2/M cell cycle phases, and chromatin immunoprecipitation (ChIP) assays were performed to follow recruitment of many chromatin regulators. We surprisingly find that subunits of the INO80, SWR-C, NuA4, SWI/SNF and RSC enzymes are primarily recruited outside of G1 phase, with the key NHEJ factor Ku70 inhibiting the recruitment of each of these enzymes in G1 cells. Furthermore, we find that recruitment of all chromatin regulators requires DSB processing and the Rad51 recombinase. In contrast to previous reports, we find that γH2AX has no significant role in the recruitment of chromatin regulators to DSBs in either G2/M or asynchronous cells, though our data do suggest that chromatin regulators may enhance γH2AX dynamics during the HR process. Recruitment of chromatin regulators is cell cycle regulated We use an established yeast system that has proven invaluable for monitoring the DSB recruitment of repair factors and chromatin regulators by ChIP analyses. This system allows for a single, persistent DSB to be induced on chromosome III by galactose-dependent expression of the HO endonuclease in a yeast strain that lacks homologous donor sequences [20] ( hmlΔhmrΔ ; Fig. 1a ). To investigate whether recruitment of chromatin regulators might be linked to the NHEJ or HR repair pathways, cells were first synchronized in G1 phase with alpha factor (αF) mating pheromone, and then released into three different media conditions: (1) galactose and αF, to induce a DSB in G1 cells; (2) galactose and hydroxyurea, to induce a DSB, as cells exit G1 phase and arrest in S phase; and (3) galactose and fresh media, to induce a DSB, as cells exit G1 and subsequently arrest at the G2/M DNA-damage checkpoint. Cell cycle arrest was confirmed by flow-cytometry analysis ( Supplementary Fig. S1a ). In this initial study, we followed recruitment of the Arp5 subunit of the INO80 chromatin remodelling enzyme. Surprisingly, recruitment of Arp5 was very low in G1 cells and in cells arrested in S phase. In contrast, Arp5 recruitment was robust in cells that had received a DSB outside of G1 phase and accumulated at the G2/M cell cycle checkpoint ( Fig. 1b ). To further investigate these results, cells were arrested in either G1 phase with αF or in G2/M with nocodazole, followed by galactose addition to induce a DSB. Initial cell cycle arrest was confirmed by flow cytometry ( Supplementary Fig. S2a ). Once again, recruitment of INO80, monitored by both Arp5 and the catalytic Ino80 subunit, was robust only when a DSB was induced in G2/M cells, with low levels of recruitment observed at a DSB induced in G1 cells ( Fig. 1c and Supplementary Fig. S2c ). Consistent with previous findings in asynchronous cultures [18] , [19] , [21] , recruitment of INO80 in G2/M-arrested cultures as well as asynchronous cultures was observed within a 10-kb chromatin domain adjacent to the DSB, and recruitment continued for at least 4 h after DSB formation ( Fig. 1c and Supplementary Fig. S2g ). Importantly, recruitment of the NHEJ factor yKu70 was also monitored, and in this case DSB recruitment was equal in both G1 and G2/M cells, similar to previous studies [7] , [12] ( Supplementary Fig. S2f ). 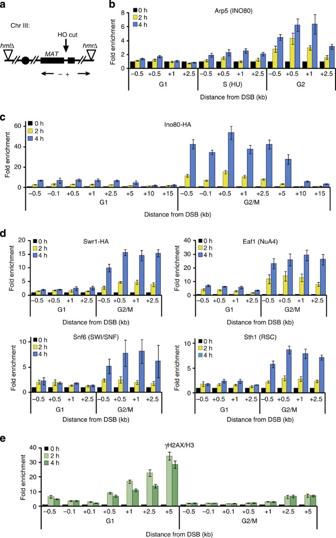Figure 1: Cell cycle-regulated recruitment of chromatin-modifying enzymes to an induced DSB. (a) Schematic of chromosome III of a donorless yeast strain harbouring a galactose-inducible HO endonuclease. Primers used during ChIP analyses are indicated according to their distance from the DSB, and designated with a ‘−’ for centrosomal proximal and ‘+’ for centrosomal distal. (b) A wild-type, donorless strain was arrested in G1 using αF and then split into three cultures: maintained in αF-arrest (‘G1’), released into fresh media containing 0.2 M hydroxyurea (‘S(HU)’) or released into fresh media alone (‘G2’). Galactose was also added at this time to induce a single DSB. Arp5 recruitment to areas surrounding the HO cut site was monitored by ChIP. (c,d) A wild-type, donorless strain was arrested with either αF (‘G1’) or nocodazole (‘G2/M’), after which a DSB was induced by addition of galactose for the indicated times. Recruitment of various chromatin remodelling complexes to the DSB region was monitored by ChIP using antibodies to the indicated enzyme subunit. Fold enrichment reflects the %IP values normalized to theACT1locus, relative to time zero values. (e) H2A phosphorylation (γH2AX) is cell cycle regulated. Cells were treated as inc, and levels of γH2AX were determined and normalized to levels of histone H3 also determined by ChIP. Data shown represent at least two biological replicates; error bars represent s.e.m. Figure 1: Cell cycle-regulated recruitment of chromatin-modifying enzymes to an induced DSB. ( a ) Schematic of chromosome III of a donorless yeast strain harbouring a galactose-inducible HO endonuclease. Primers used during ChIP analyses are indicated according to their distance from the DSB, and designated with a ‘−’ for centrosomal proximal and ‘+’ for centrosomal distal. ( b ) A wild-type, donorless strain was arrested in G1 using αF and then split into three cultures: maintained in αF-arrest (‘G1’), released into fresh media containing 0.2 M hydroxyurea (‘S(HU)’) or released into fresh media alone (‘G2’). Galactose was also added at this time to induce a single DSB. Arp5 recruitment to areas surrounding the HO cut site was monitored by ChIP. ( c , d ) A wild-type, donorless strain was arrested with either αF (‘G1’) or nocodazole (‘G2/M’), after which a DSB was induced by addition of galactose for the indicated times. Recruitment of various chromatin remodelling complexes to the DSB region was monitored by ChIP using antibodies to the indicated enzyme subunit. Fold enrichment reflects the %IP values normalized to the ACT1 locus, relative to time zero values. ( e ) H2A phosphorylation (γH2AX) is cell cycle regulated. Cells were treated as in c , and levels of γH2AX were determined and normalized to levels of histone H3 also determined by ChIP. Data shown represent at least two biological replicates; error bars represent s.e.m. Full size image Given the unanticipated result of differential recruitment of INO80 during the cell cycle, we conducted further ChIP assays to monitor recruitment of several other chromatin regulators, including subunits of the SWR-C, SWI/SNF and RSC remodelling enzymes, as well as the NuA4 histone acetyltransferase complex. Interestingly, the recruitment of each of these chromatin regulators was much more robust outside of G1 phase, compared with G1-arrested cells ( Fig. 1d and Supplementary Fig. S2d ). These data suggest that there may be a common, cell cycle-regulated mechanism for recruitment of multiple chromatin regulators to a DSB. γH2AX is dispensable for recruitment of chromatin regulators Previous ChIP studies have indicated that formation of γH2AX is required for efficient DSB recruitment of INO80 and SWR-C within asynchronous cell populations [18] , [19] . To understand how this mechanism interfaces with cell cycle regulation, we monitored the levels of γH2AX in chromatin surrounding DSBs formed in our experiments. Surprisingly, the levels of γH2AX surrounding the DSB were much lower in cells outside of G1 compared with those arrested in G1 ( Fig. 1e and Supplementary Figs S1b and S3a ). These contrasting levels of γH2AX are not due to changes in nucleosome density, as levels of H3 and H2B were reduced only approximately twofold in G2/M samples compared with G1, presumably due to DSB processing ( Supplementary Fig. S3d , see below). Levels of γH2AX were also reduced in G2/M samples at early time points after DSB induction, when end processing has not progressed significantly (for example, 30′), and when ChIP samples were processed in buffers containing 0.5 M NaCl ( Supplementary Fig. S3b,c ). Furthermore, we monitored formation of γH2AX following exposure of synchronized cells to the DSB-inducing agent phleomycin and again observed more robust γH2AX formation in G1 cells compared with G2/M cells, indicating that these cell cycle differences are not unique to an HO-induced DSB ( Supplementary Fig. S3e,f ). The data suggest that γH2AX levels or dynamics may be dramatically altered in chromatin surrounding DSBs formed within G2/M cells. Furthermore, these results imply that the levels of γH2AX and chromatin regulators are anti-correlated, indicating that γH2AX may not be involved in their recruitment. To re-examine the role of γH2AX in recruitment of chromatin regulators, we monitored recruitment events in two different strains that lack γH2AX: a strain expressing a derivative of H2A (bulk yeast H2A is the equivalent to mammalian H2A.X) where serine 129 has been changed to an alanine residue ( hta1,2-S129A ) [22] , and a strain expressing a truncated H2A derivative that removes the final four C-terminal amino acids, including the Mec1/Tel1 phosphorylation site ( hta1,2-S129Δ4 ) [23] . Importantly, both of these strains exhibited similar sensitivity to the DNA-damaging agent methyl methanesulfonate, as expected from previous studies [24] ( Supplementary Fig. S4a ). Surprisingly, neither H2A-S129A nor H2A-S129Δ4 reduced INO80 recruitment, irrespective of whether a DSB was induced in asynchronous or G2/M-arrested cells ( Fig. 2a and Supplementary Fig. S4c ). Indeed, recruitment of the Arp5 subunit of INO80 was slightly elevated in the strain expressing the C-terminal H2A truncation ( Fig. 2a ). Similar results were found for Sth1 (RSC), Eaf1 (NuA4), Eaf3 (NuA4/Rpd3), Swi2 (SWI/SNF) and Yaf9 (NuA4/SWR-C) ( Fig. 2b and Supplementary Fig. S4d,e ). Interestingly, however, recruitment of the Snf6 subunit of SWI/SNF complex was markedly decreased in the absence the H2A C-terminus, even though its recruitment is not affected by the H2A-S129A substitution (compare Fig. 2b and Supplementary Fig. S4e ), implicating other residues within the H2A C-terminus. Why recruitment of the Swi2 and Snf6 subunits of SWI/SNF differentially respond to the H2A C-terminus remains unclear. However, when taken together, the data indicate that γH2AX does not regulate recruitment of chromatin regulators. 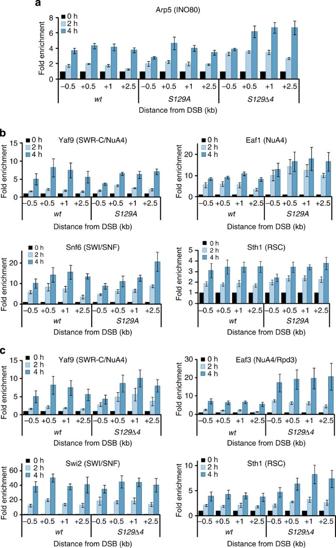Figure 2: γH2AX is not essential for recruitment of chromatin regulators to a DSB. (a–c) Isogenic, donorless wild-type (wt),hta1,2-S129A(S129A) andhta1,2-S129Δ4(S129Δ4) strains were arrested in G2/M using nocodazole and analysed by ChIP for recruitment of the indicated chromatin-modifying enzyme subunits to the DSB region at the indicated time points after DSB induction. Data shown represent at least two biological replicates; error bars represent s.e.m. Figure 2: γH2AX is not essential for recruitment of chromatin regulators to a DSB. ( a – c ) Isogenic, donorless wild-type ( wt ), hta1,2-S129A ( S129A ) and hta1,2-S129Δ4 ( S129Δ4 ) strains were arrested in G2/M using nocodazole and analysed by ChIP for recruitment of the indicated chromatin-modifying enzyme subunits to the DSB region at the indicated time points after DSB induction. Data shown represent at least two biological replicates; error bars represent s.e.m. Full size image Although our hta1,2-S129Δ4 and hta1,2-S129A alleles were created within the same JKM strain background as two previously published studies, our ChIP data are contradictory [18] , [19] . We obtained the previously published hta1,2-S129* strain (also a four residue truncation; GA2824 (ref. 18 )) and found that this strain shows similar sensitivity to DNA-damaging agents as our hta1,2-129Δ4 strain ( Supplementary Fig. S4a ). However, strain GA2824 also exhibits an unexpected, severe growth defect in raffinose or lactate media, and liquid cultures arrested growth at low cell densities (for example, OD 600 =0.4). Flow-cytometry analysis also demonstrates that asynchronous cultures of GA2824 grown in raffinose media accumulate in the G1 phase of the cell cycle, and furthermore, this cell cycle distribution does not change following galactose addition to induce the HO endonuclease ( Supplementary Fig. S4b ). These growth defects precluded our ability to obtain high-quality, reproducible ChIP data with this strain. Previous studies with the GA2824 strain have also indicated that γH2AX is required for efficient DSB processing [18] . However, a recent study shows that γH2AX inhibits DSB processing [25] , and we also observe increased levels of RPA adjacent to a DSB in our hta1,2-S129Δ4 and hta1,2-S129A strains ( Supplementary Fig. S4f ), consistent with a negative role for γH2AX in DSB processing. Because DSB processing is restricted in G1 cells, and INO80 and SWR-C are also poorly recruited in G1 cells, it seems likely that the aberrant slow growth and G1 accumulation phenotypes of the GA2824 strain were the cause of the previously observed defects in both DSB end processing and chromatin regulator recruitment, rather than a lack of γH2AX [18] . Chromatin regulator recruitment requires DNA-end processing Our results indicate that the cell cycle regulation of the DSB response has a key role in the recruitment of chromatin regulators to the DSB. Recruitment of chromatin factors outside of G1 coincides with the binding of RPA to single-stranded DNA (ssDNA) that is formed by the extensive processing of the DSB by the redundant Sgs1/Dna2 and Exo1 resection pathways [5] , [26] , [27] , [28] ( Supplementary Fig. S2d ). Notably, this relationship is also consistent with the poor recruitment of Arp5 (INO80) to a DSB induced within HU-treated cells ( Fig. 1b ), as HU activates cell cycle checkpoints that inhibit DSB processing [29] . To examine the possibility that DSB recruitment of chromatin regulators requires resection, we monitored recruitment in isogenic sgs1Δ , exo1Δ and sgs1Δexo1Δ strains. Strikingly, recruitment of Arp5 (INO80), Snf6 (SWI/SNF), Sth1 (RSC), Eaf3 (NuA4/Rpd3) or Yaf9 (NuA4/SWR-C) was greatly reduced in the sgs1Δexo1Δ double mutant, with significant reductions occurring 500 bp distal to the DSB and reducing to basal levels by 2.5 kb distal ( Fig. 3a ). Importantly, the sgs1Δexo1Δ strain showed a cell cycle profile identical to the wild-type strain ( Supplementary Fig. S5a ). Consistent with the functional redundancy of these processing enzymes, only a minor defect in recruitment of INO80 to a DSB was observed in exo1Δ or sgs1Δ single mutants ( Supplementary Fig. S5b ). Interestingly, γH2AX levels were also increased in the double mutant, most notably distal from the break ( Fig. 3b ). These results suggest that DSB processing is required for optimal recruitment of multiple chromatin regulators and that their recruitment correlates with decreased γH2AX levels. 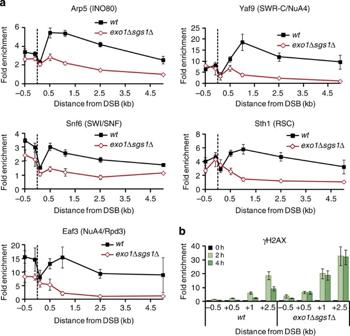Figure 3: DNA-end processing is required for recruitment to a DSB. Isogenic, donorless wild-type (wt) andexo1Δsgs1Δstrains were grown asynchronously and analysed by ChIP in the region surrounding the DSB for (a) recruitment of the indicated chromatin-modifying enzyme subunits 4 h after induction (dotted line indicates the HO cut site) and (b) levels of γH2AX at the indicated time points after induction. Data shown represent at least two biological replicates; error bars represent s.e.m. Figure 3: DNA-end processing is required for recruitment to a DSB. Isogenic, donorless wild-type ( wt ) and exo1Δsgs1Δ strains were grown asynchronously and analysed by ChIP in the region surrounding the DSB for ( a ) recruitment of the indicated chromatin-modifying enzyme subunits 4 h after induction (dotted line indicates the HO cut site) and ( b ) levels of γH2AX at the indicated time points after induction. Data shown represent at least two biological replicates; error bars represent s.e.m. Full size image Previous studies have shown that the Ku70/80 heterodimer inhibits DSB processing in G1 cells, limiting DNA-end resection and promoting NHEJ [7] . In addition, loss of Ku70 allows Rad52- and Rad51-dependent recombination events to occur efficiently in G1-arrested cells [30] . To test whether the decreased recruitment of chromatin factors in G1 is due to limited DSB processing, an yku70Δ strain was arrested in G1, and ChIP assays were performed at an HO-induced DSB. Strikingly, recruitment of all chromatin regulators was restored to high levels in the G1-arrested yku70Δ cells ( Fig. 4a ). In contrast, γH2AX levels were reduced in the G1-arrested yku70Δ strain to levels previously seen in G2/M cultures, once again displaying an inverse relationship to the recruitment of chromatin regulators ( Fig. 4b ). These results suggest that yKu70/80 inhibits recruitment of chromatin regulators in G1 cells, and furthermore, that recruitment is independent of cell cycle position. Notably, inactivation of Ku70 does not restore the recruitment of INO80 and SWI/SNF in the absence of Sgs1 and Exo1 ( Supplementary Fig. S5d ), strongly supporting the idea that DSB processing facilitates the recruitment of chromatin-regulatory factors at the DSB. 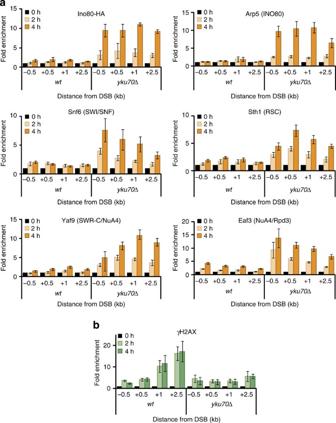Figure 4: Ku inhibits recruitment of chromatin regulators in G1. Isogenic, donorless wild-type (wt) andyku70Δstrains were arrested in G1 with αF and analysed by ChIP for (a) recruitment of the indicated chromatin-modifying enzyme subunits and (b) levels of γH2AX in the DSB region at the indicated time points after DSB induction. Data shown represent at least two biological replicates; error bars represent s.e.m. Figure 4: Ku inhibits recruitment of chromatin regulators in G1. Isogenic, donorless wild-type ( wt ) and yku70Δ strains were arrested in G1 with αF and analysed by ChIP for ( a ) recruitment of the indicated chromatin-modifying enzyme subunits and ( b ) levels of γH2AX in the DSB region at the indicated time points after DSB induction. Data shown represent at least two biological replicates; error bars represent s.e.m. Full size image Previous work has shown that the yeast Mre11/Rad50/Xrs2 (MRX) complex directs processing of the initial ~100 bp of DNA proximal to the DSB [28] . Indeed, we find high levels of the ssDNA-binding protein RPA proximal to the DSB in sgs1Δexo1Δ cells ( Supplementary Fig. S5c ), a result consistent with MRX-dependent resection. To test whether MRX-dependent processing might be responsible for the residual recruitment of chromatin regulators observed in the sgs1Δexo1Δ double mutant, Arp5 (INO80) recruitment was monitored in wild-type and mre11Δ cells arrested in G2/M. Note that a sgs1Δexo1Δmre11Δ strain was not constructed due to the expected growth defects of this strain. As shown in Supplementary Fig. S5e , Arp5 (INO80) recruitment was lost from DSB proximal chromatin in the absence of Mre11, and overall levels are similar to those found in G1 cells. Taken together, these data suggest a model in which DSB processing controls the recruitment of chromatin regulators, either through direct interactions with ssDNA or by subsequent events of the HR or the DNA-damage checkpoint signalling pathway. Rad51 is required for recruitment of chromatin regulators Following DSB processing, the ssDNA ends are initially bound by the ssDNA-binding protein RPA, which is subsequently replaced by the key recombinase, Rad51 (ref. 31 ). Therefore, we tested whether Rad51 is key for recruitment of chromatin regulators. Strikingly, recruitment of Arp5 (INO80) was nearly eliminated in the G2/M-arrested rad51Δ strain, with a reduction to the twofold recruitment level seen in G1 cells ( Fig. 5a ). Furthermore, recruitment of Swi2 (SWI/SNF), Snf6 (SWI/SNF), Sth1 (RSC), Eaf3 (NuA4/Rpd3) and Yaf9 (NuA4/SWR-C) were also nearly abolished ( Fig. 5a and Supplementary Fig. S6a ). In addition, levels of γH2AX were also increased in the absence of Rad51, consistent with one or more chromatin regulators controlling γH2AX dynamics ( Fig. 5c ). Importantly, Rad51 is not required for DSB processing or establishing the checkpoint response [28] , [31] , [32] ( Supplementary Fig. S6b ), indicating that formation of ssDNA is not sufficient for recruitment of chromatin regulators or for decreased levels of γH2AX. 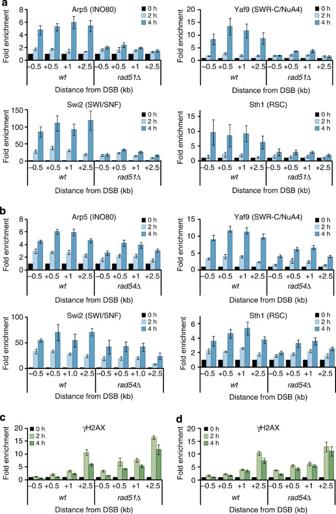Figure 5: Rad51 is necessary for recruitment of chromatin regulators. Isogenic, donorless wild-type (wt) and (a)rad51Δor (b)rad54Δstrains were arrested in G2 with nocodazole and analysed by ChIP for recruitment of the indicated chromatin-modifying enzyme subunits to the region the DSB region at the indicated time points after DSB induction. A dotted line indicates the HO cut site. (c,d) Levels of γH2AX determined by ChIP in the DSB region of experiments described inaandb, respectively. Data shown represent at least two biological replicates; error bars represent s.e.m. Figure 5: Rad51 is necessary for recruitment of chromatin regulators. Isogenic, donorless wild-type ( wt ) and ( a ) rad51Δ or ( b ) rad54Δ strains were arrested in G2 with nocodazole and analysed by ChIP for recruitment of the indicated chromatin-modifying enzyme subunits to the region the DSB region at the indicated time points after DSB induction. A dotted line indicates the HO cut site. ( c , d ) Levels of γH2AX determined by ChIP in the DSB region of experiments described in a and b , respectively. Data shown represent at least two biological replicates; error bars represent s.e.m. Full size image Formation of the Rad51-ssDNA nucleoprotein filament has a key role in the subsequent search and capture of a homologous DNA duplex. Rad51 also recruits Rad54 that is a member of the Snf2/Swi2 family of ATPases and exhibits weak chromatin remodelling activity in vitro [33] . Rad54 has at least two roles during HR. First, Rad54 has an ATP-independent activity that facilitates Rad51 loading onto DNA proximal to the DSB [34] , [35] , and second, Rad54 has an ATP-dependent role to convert the initial joint molecule into a stable, strand-invasion product that can be extended by DNA polymerases [35] , [36] . To investigate possible roles for Rad54 in the recruitment of chromatin regulators, a DSB was induced in G2/M-arrested rad54Δ or rad54 K341R strains, the latter of which contains an allele of RAD54 that inactivates its ATPase activity [37] . ChIP assays for Arp5 (INO80), Swi2 (SWI/SNF), Sth1 (RSC), Eaf3 (NuA4/Rpd3) or Yaf9 (NuA4/SWR-C) indicate a small but reproducible role for Rad54. In all of these cases, there is a defect in recruitment at locations proximal to the DSB, but less of an effect at distal locations ( Fig. 5b and Supplementary Fig. S7a ). However, very few recruitment defects were observed in the strain harbouring the ATPase-defective version of Rad54 ( Supplementary Fig. S7b ). In contrast, recruitment of Snf6 (SWI/SNF) was nearly abolished in the absence of Rad54, or when the ATPase activity of Rad54 was inactivated ( Supplementary Fig. S7 ). Thus, recruitment of the Snf6 subunit of SWI/SNF is distinct from both the Swi2 catalytic subunit and other chromatin regulators, requiring both Rad51 and the ATPase activity of Rad54. We have shown here that the recruitment of at least five chromatin-regulatory enzymes—INO80, SWR-C, SWI/SNF, RSC and NuA4—are recruited to a DNA DSB in a cell cycle-dependent manner, with at least five-fold higher levels observed in G2/M cells compared with G1 cells. Our results indicate that recruitment is inhibited in G1 cells by the Ku70/80 complex, and that robust recruitment outside G1 is promoted by early steps of the HR process that lead to formation of the Rad51 nucleoprotein filament. Our data are not inconsistent with roles for chromatin regulators during NHEJ, as recruitment of chromatin regulators is low but not entirely abolished in G1. Indeed, recruitment of the INO80 complex in G1 cells is not affected by loss of Rad51, suggesting an independent mode for recruitment of chromatin regulators at this cell cycle phase. However, Rad51 is at least partially required for recruitment of INO80 in G1 cells that lack Ku70 ( Supplementary Fig. S6c ). Our data strongly support the view that chromatin regulators primarily impact repair events such as HR that occur following S phase. This idea is consistent with the known roles for the RSC, SWI/SNF, INO80 and SWR-C remodelling enzymes in distinct steps of HR and in cell cycle-checkpoint control [22] , [38] , [39] , [40] , [41] . Although recruitment of human INO80 to DSBs does not require γH2AX [42] , three studies previously implicated γH2AX in the recruitment of the yeast INO80 and SWR-C remodelling enzymes [18] , [19] , [21] . This conclusion was based primarily on three results: (1) ChIP assays using a strain harbouring an H2A C-terminal truncation allele ( hta1,2-S129Δ4 ); (2) ChIP assays in a mec1 tel1 double mutant; and (3) co-purification of INO80 with γH2AX from cells treated with DNA-damaging agents. Our current data indicate that the interpretation of previous ChIP data was confounded by the cell cycle distribution of the strain used: the previously employed H2A-S129 Δ 4 strain exhibits an aberrant accumulation of cells in G1, conditions where recruitment of INO80 and SWR-C is poor. Likewise, we envision that the lack of G2 checkpoint arrest in the mec1 tel1 double mutant led to a similar issue. Furthermore, we note that purification of INO80 in low salt buffers leads to co-purification of all four core histones [21] , so it is expected that some level of γH2AX will be associated with INO80 under DNA-damage conditions. It is perhaps not surprising that γH2AX does not control recruitment of INO80 or SWR-C, because their recruitment requires hours, whereas formation of the γH2AX domain occurs within minutes. In addition, loss of γH2AX leads to relatively little sensitivity to DNA-damaging agents, whereas inactivation of INO80 causes a strong impact on the DNA-damage response [18] , [24] . Furthermore, as shown here and previously, the chromatin distribution of γH2AX and INO80 do not coincide at DSBs [16] , [19] , and furthermore, our ChIP data show an anti-correlation in the recruitment of chromatin regulators and γH2AX signal. Although it remains a possibility that γH2AX may have a role within G1 cells, our data do not support a dominant role of γH2AX in recruitment of chromatin regulators to DSBs. Previous studies in budding yeast have demonstrated high levels of γH2AX in both asynchronous cell populations and cells arrested in G1. However, no previous studies have reported γH2AX levels for DSBs induced in cells synchronized outside of G1 phase. We were quite surprised to find a dramatic decrease in γH2AX levels for DSBs induced with G2/M cells. This decrease does not appear to be due solely to DSB processing, as γH2AX levels remain high in rad51Δ cells where DSB resection occurs normally. We envision that γH2AX may be established at normal levels in G2/M cells, but that it is subjected to enhanced dynamics, likely catalysed by one or more chromatin regulators. One possibility is that the low levels of γH2AX reflect dynamic exchange of H2A for H2A.Z by the SWR-C complex [22] , [43] , [44] , although we find that γH2AX levels are not increased in a G2/M-arrested swr1Δ strain ( Supplementary Fig. S8 ). Removal of γH2AX, particularly in G2/M cells, is consistent with recent studies and our own data, indicating a negative impact of γH2AX on DSB processing [25] ( Supplementary Fig. S4f ). We note that, while all the chromatin-modifying complexes examined share a common set of requirements for recruitment to a DSB, only the Snf6 subunit of SWI/SNF shows a strong requirement for both the H2A C-terminus and Rad54, though neither was needed to recruit the Swi2 catalytic subunit. Our previous study indicated that Snf6 is uniquely associated with SWI/SNF [45] , so it seems unlikely that it is recruited to DSBs by an independent mechanism. We favour a model in which the Snf6 subunit does not directly associate with nucleosomal DNA, and thus its crosslinking during the ChIP procedure is highly sensitive to small changes in SWI/SNF chromatin interactions. How might Rad51 control the recruitment of chromatin regulators? One simple possibility is that the Rad51-ssDNA filament functions as an assembly platform for chromatin regulators and that each of these enzymes may directly interact with Rad51. Although there are no subunits held in common among all of the chromatin regulators that we have monitored, we note that each enzyme does harbour a member of the actin-related protein (ARP) family that may provide a common interaction surface [46] . Alternatively, it is possible that only a limited number of regulators interact directly with Rad51, and the activity of these few enzymes control recruitment of other complexes. Testing this latter possibility may require the development of strains where multiple essential regulators can be removed simultaneously. Recently, studies in Drosophila and yeast have demonstrated that DSB processing and the Rad51 recombinase are required for long-range, intra-nuclear movements of DSB chromatin during the homology search step of HR [40] , [47] , and to regulate repair of heterochromatic DSBs by HR [48] . Interestingly, yeast studies indicate that the ATPase activity of Rad54 is also essential for enhanced DSB mobility [47] . Although the INO80 enzyme has been suggested as a candidate factor that catalyses DSB mobility [41] , our recruitment data suggests that other remodelling enzymes may also contribute, as all enzymes tested require Rad51 for their recruitment to DSBs. How ATP-dependent remodelling might promote chromosome dynamics is currently unclear, though the orchestration of such a complex event may provide one explanation for why so many chromatin regulators are recruited to a DSB. Yeast strains All strains are derivatives of JKM139 or JKM179 (ref. 20 ) and were generated by the one-step PCR disruption method. Disruptions were confirmed by PCR analysis. Full genotypes are available in Supplementary Table S1 . All strains were grown at 30 °C in lactate media (1% yeast extract, 2% bactopeptone, 2% lactic acid, 3% glycerol and 0.05% glucose, pH 6.6) or YPR (1% yeast extract, 2% bactopeptone and 2% raffinose) pre-induction. HO induction was achieved by adding 2% galactose to each culture. Cultures were arrested in G1 using 1 μM αF treatment for 4 h ( bar1Δ strains). G2/M arrest was achieved using 30 μg ml −1 nocodazole for 4–5 h. Arrests were confirmed by visual microscopy, followed by budding indices. Chromatin immunoprecipitation ChIPs were performed with some modifications as previously described [49] : 50 ml of mid-log phase cells were cross-linked by adding 1% (final) formaldehyde for 15 min at room temperature, followed by neutralization with 150 mM (final) glycine for 5 min. Cell pellets were washed twice in cold TBS (50 mM Tris-Cl, pH 7.5, and 150 mM NaCl) and then resuspended in cold 400 μl FA-lysis buffer (50 mM HEPES-KOH, pH 7.5, 140 mM NaCl, 1 mM EDTA, 1% Triton X-100 and 0.1% sodium deoxycholate) plus 1 × fresh ‘complete’ protease inhibitor cocktail (PIC; Roche). Cells were lysed with an equal volume of glass beads at 4 °C. After glass bead removal, samples were sonicated to shear DNA to an average size of 500 bp. An additional 1 ml FA-lysis buffer plus PIC was added, and the chromatin lysate was purified by centrifugation at 14,000 r.p.m. for a total of 1.5 h at 4 °C. For most IPs, 100–200 μl of the purified chromatin lysate was diluted up to 400 μl with FA-lysis buffer plus PIC, and 1–2 μl antibody was added. For SWI/SNF IPs, 1% (final) sarkosyl was also added. For high-salt γH2AX IPs, FA-lysis buffer was replaced by FA-500 buffer (50 mM HEPES-KOH, pH 7.5, 500 mM NaCl, 1 mM EDTA, 1% Triton X-100 and 0.1% sodium deoxycholate) All IPs were incubated overnight at 4 °C, followed by incubation with 15 μl equilibrated sepharose protein A beads (50% slurry; Rockland) for 2 h at 4 °C. Pelleted beads were washed at room temperature, for 5–10 min each, sequentially with FA-lysis buffer (except high-salt γH2AX IPs), FA-500 buffer, LiCl wash buffer (10 mM Tris-Cl, pH 8.0, 250 mM LiCl, 1 mM EDTA, 0.5% NP-40 and 0.5% sodium deoxycholate) and Tris-EDTA (10 mM Tris-Cl, pH 7.5, and 1 mM EDTA), followed by elution in Elution buffer (50 mM Tris-Cl, pH 7.5, 10 mM EDTA and 1% SDS) shaking for 10 min at 65 °C. For input samples, 10 μl purified chromatin lysate was diluted in 450 μl Tris-EDTA. All samples (IPs and inputs) were treated with proteinase K (0.2 mg ml −1 final) at 42 °C for 2 h, cross-links reversed by incubation at 65 °C for ≥5 h, and purified by phenol-chloroform extraction and ethanol precipitation. Input samples were diluted 20 × over IP samples during DNA purification. The immunoprecipitated and input DNA was analysed by quantitative real-time PCR with iTaq SYBR Green Supermix with ROX (Bio-Rad). Primer sequences are available in Supplementary Table S2 . Fold enrichment represents the ratio of recovered DNA to input DNA of the break region, normalized to the same ratio obtained for the ACT1 open reading frame. These ratios were additionally normalized to pre-induction (0 h) values and corrected for DSB induction. Percent IP (for anti-RPA only) represents the ratio of immunoprecipitated DNA to input DNA corrected for dilution, and is not normalized to a control region, because those values approached zero. Error bars indicate s.e.m. from at least two independent biological replicas and four PCR reactions. Western blotting Whole-cell extracts were prepared by trichloroacetic acid precipitation, and proteins were separated by SDS–polyacrylamide gel electrophoresis in 18% acrylamide gels. Samples were blotted onto polyvinylidene difluoride membranes and probed with antibodies using standard methods. Antibodies Rabbit polyclonal antibodies to HA tag (ab9110), Arp5 (ab12099), Yaf9 (ab4468), Eaf3 (ab4467) and H2A-S129phos (γH2AX; ab15083) are commercially available from Abcam. Anti-H2B (39237) is available from Active Motif. Anti-Snf6 and anti-Swi2, anti-RPA, anti-Sth1, anti-Eaf1 and anti-Ku antibodies were kind gifts from J. Reese (Pennsylvania State University), V. Borde (Institut Curie), B. Cairns (University of Utah), J. Cote (Laval University Cancer Research Center) and S.E. Lee (University of Texas Health Science Center at San Antonio), respectively. Flow cytometry Approximately 1 ml of mid-log phase (~1–2 × 10 7 ) cells were collected per sample, washed in water, fixed in 100% ethanol and incubated at 4 °C rocking overnight. After fixation, cells were again washed in water, resuspended in 50 mM Tris, pH 8.0, containing 200 μg ml −1 RNase A, and incubated at 37 °C for 2–4 h. Samples were then pelleted and resuspended in 50 mM Tris pH 7.5 containing 2 mg ml −1 Proteinase K and incubated at 50 °C for 30–60 min, followed by resuspension in 500 μl FACS buffer (200 mM Tris, pH 7.5, 200 mM NaCl and 78 mM MgCl 2 ). Approximately 100 μl of each sample was then incubated for 10 min at room temperature with 1 ml Sytox solution (50 mM Tris, pH 7.5 and 1 μM Sytox Green (Molecular Probes; S-7020)) and sonicated gently for approximately 30 s directly before analysis on a BD FACSCalibur flow cytometer. Data analysis and preparation was completed with FlowJo. How to cite this article: Bennett, G. et al. DNA repair choice defines a common pathway for recruitment of chromatin regulators. Nat. Commun. 4:2084 doi: 10.1038/ncomms3084 (2013).